Structural insights into protein-only RNase P complexed with tRNA RNase P is the essential activity removing 5′-leader sequences from transfer RNA precursors. RNase P was always associated with ribonucleoprotein complexes before the discovery of protein-only RNase P enzymes called PRORPs (PROteinaceous RNase P) in eukaryotes. Here we provide biophysical and functional data to understand the mode of action of PRORP enzymes. Activity assays and footprinting experiments show that the anticodon domain of transfer RNA is dispensable, whereas individual residues in D and TψC loops are essential for PRORP function. PRORP proteins are characterized in solution and a molecular envelope is derived from small-angle X-ray scattering. Conserved residues are shown to be involved in the binding of one zinc atom to PRORP. These results facilitate the elaboration of a model of the PRORP/transfer RNA interaction. The comparison with the ribonucleoprotein RNase P/transfer RNA complex suggests that transfer RNA recognition by PRORP proteins is similar to that by ribonucleoprotein RNase P. RNase P is the ubiquitous activity that catalyses the 5′-maturation of transfer RNAs (tRNAs), as well as of a number of other substrates such as ribosomal RNA, messenger RNA, transfer-messenger RNA or riboswitches [1] , [2] , [3] . RNase P was first described in bacteria where it is composed by a ribonucleoprotein (RNP) complex whose RNA component (P RNA) holds the catalytic activity [4] . RNP RNase P was later found in all three main branches of life, that is, Bacteria, Archaea and Eukarya, and was thus believed to occur universally as a RNP complex [5] . This concept was challenged by early experiments in human mitochondria and spinach chloroplasts that suggested that another type of RNase P devoid of RNA component existed in these organelles [6] , [7] . Still the dogma of the universality of RNP RNase P remained until the recent characterization of a novel type of RNase P in human mitochondria and plant organelles [8] , [9] . This novel variant is composed of a single protein that we called PRORP (for PROteinaceous RNase P) and occurs in nearly all major phyla of eukaryotes [9] . Furthermore, RNP RNase P has not been retained in all organisms because, in both Arabidopsis and Trypanosoma , PRORP enzymes were found to support RNase P activity in both organelles and the nucleus [10] , [11] . The discovery of PRORP enzymes leads to the question of the respective mode of action of RNP and protein enzymes catalysing the same reaction. RNP RNase P activity is well characterised [2] , [12] , in particular, recent advances such as the determination of the three-dimentional structure of a bacterial RNase P in complex with tRNA have been very important developments [13] . Substrate recognition by RNP RNase P involves the binding to regions distant from the actual cleavage site. It includes stacking interactions between bases in the D and TψC loops of tRNAs and the P RNA specificity (S) domain, an A-minor interaction at the acceptor stem and the formation of canonical base pairs at the 3′-end of tRNA. In particular, key interactions take place between the unstacked bases G19 and C56 of tRNA and the S domain of RNase P. It is also notable that no interaction takes place with the anticodon arm of tRNA. The catalytic active site of RNP RNase P is composed of phosphate backbone moieties, a conserved uridine and at least two catalytically important metal ions [13] . In contrast, the mode of action of PRORP proteins is unknown. These protein-only RNase P enzymes are characterized by the presence of pentatricopeptide (PPR) repeats [14] in their N-terminal part that are believed to be involved in RNA binding and possess an upstream zinc-finger-like motif. The most conserved part of PRORP enzymes lies in their C-terminal part. This region was predicted to be a metallonuclease domain [8] and consigns PRORP to the large family of PIN-like/NYN (N4BP1, YacP-like Nuclease) domain putative ribonucleases [15] . Initial comparison of PRORP and RNP RNase P has suggested that the two classes of enzymes share common features. They both appear to require Mg 2+ for phosphodiester hydrolysis and both generate 5′-phosphate and 3′-hydroxyl products [8] . However, studies using spinach chloroplast extracts and recombinant Arabidopsis PRORP have shown that PRORP is a fundamentally different catalyst than RNP RNase P. The replacement of the phosphodiester backbone of a precursor tRNA by a phosphorothioate moiety at the level of the 5′-maturation site resulted in a strong inhibition of bacterial RNase P activity, while PRORP activity was unaltered [16] , [17] . To gain functional insight into this novel type of RNase P activity, we investigated how Arabidopsis PRORP1 binds tRNA substrates and we performed a biophysical characterization of PRORP1 and 2. This enabled us to define initial mechanistic data on PRORP mode of action. The proposed mode of RNA recognition by PRORP shows striking similarity with that of RNP RNase P, which suggests that protein-only RNase P might have converged to the same tRNA-binding strategy as RNP RNase P. tRNA cis elements required for PRORP activity To get mechanistic insights into the mode of action, in particular of RNA recognition of PRORP enzymes, we performed RNase P cleavage assays with recombinant PRORP1 and different mutants of mitochondrial tRNA Cys precursor, a known substrate of PRORP1 in vivo ( Fig. 1 ). We first removed the anticodon domain from the tRNA precursor, which did not result in significant decrease of cleavage by PRORP. Then, the removal of both the D and anticodon domains was tested. The resulting mini helix was not cleavable by PRORP. As PRORP enzymes are able to cleave the 5′-leader sequence of any tRNA of canonical structure in vitro [8] , [9] , [10] , [11] , we postulated that the determinants for tRNA recognition by PRORP must reside among positions universally conserved in tRNAs [18] . We thus applied point mutations to such positions in tRNAs to investigate their effect on PRORP activity. The mutation of G18 in the D-loop to A and C, respectively, resulted in severe impairment and total loss of RNase P activity, whereas the mutation of G19 to A or C did not affect RNase P activity. However, mutations of C56 in the TψC loop to A or G resulted in total loss of RNase P cleavage. In the same loop, mutations of G57 to A and C resulted in unaffected and total loss of PRORP cleavage, respectively, consistent with the conservation of a purine at position 57 in tRNA [18] . Next, the exchange of G-C, the first base pair of the acceptor stem by C-G did not result in decreased cleavage efficiency, although we cannot exclude that mis-cleavage did not occur. Finally, we investigated the nature of the 3′-end of tRNA precursors. The absence of a 3′-trailer sequence did not affect 5′-cleavage, whereas the occurrence of a 3′-CCA group strongly reduced RNase P activity ( Fig. 1 ). Further analyses will be necessary to determine if 3′-CCA groups act as PRORP binding antideterminants for all tRNAs, and to uncover the precise involvement of the length and the nature of residues in 3′-trailer sequences for PRORP activity. 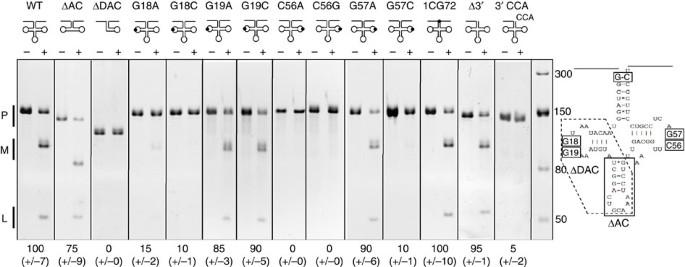Figure 1: RNase Pin vitrocleavage assays performed withArabidopsisrecombinant PRORP1 and variants of mitochondrial tRNACysprecursors. + and − indicate the absence and presence of PRORP proteins in the reactions. WT is the wild-type tRNACys, ΔAC the tRNA without the anticodon domain, and ΔDAC without both anticodon and D domains. G18A, for example, shows a tRNA where the guanosine at position 18 was mutated into an adenine. 1CG72 is a tRNA where the G-C base pair at positions 1 and 72 was swapped to a C-G. Δ3′-shows a tRNA precursor without 3′-trailer sequence and 3′-CCA, the precursor with a mature 3′-end containing a CCA. P stands for tRNA precursors, M the 5′-mature products and L the cleaved 5′-leader fragments. The molecular weights of markers are given in nucleotides. PRORP cleavage products were quantified with ImageGauge (Fujifilm). Values were normalized so that 100 corresponds to the cleavage efficiency observed for wild-type tRNACysprecursor. Cleavage efficiencies are given below the respective panels together with s.d.’s for three representative experiments. Figure 1: RNase P in vitro cleavage assays performed with Arabidopsis recombinant PRORP1 and variants of mitochondrial tRNA Cys precursors. + and − indicate the absence and presence of PRORP proteins in the reactions. WT is the wild-type tRNA Cys , ΔAC the tRNA without the anticodon domain, and ΔDAC without both anticodon and D domains. G18A, for example, shows a tRNA where the guanosine at position 18 was mutated into an adenine. 1CG72 is a tRNA where the G-C base pair at positions 1 and 72 was swapped to a C-G. Δ3′-shows a tRNA precursor without 3′-trailer sequence and 3′-CCA, the precursor with a mature 3′-end containing a CCA. P stands for tRNA precursors, M the 5′-mature products and L the cleaved 5′-leader fragments. The molecular weights of markers are given in nucleotides. PRORP cleavage products were quantified with ImageGauge (Fujifilm). Values were normalized so that 100 corresponds to the cleavage efficiency observed for wild-type tRNA Cys precursor. Cleavage efficiencies are given below the respective panels together with s.d.’s for three representative experiments. Full size image Taken together, our results show that the anticodon domain is not involved in RNA recognition by PRORP. The nature of residues at positions 1 and 72 is not discriminant for the activity, while the 3′-CCA seems to act as an antideterminant for PRORP binding. As residues at positions 18 and 57 are involved in interactions between loops D and TψC of tRNA [18] , an interaction between loops D and TψC appears to be strictly required for PRORP function. However, the conservation of the G19:C56 interaction does not appear to be critical, although the presence of a cytidine at position 56 seems to be indispensable. Thus, precise residues in loops D and TψC seem to be essential for substrate recognition by PRORP. tRNA residues in interaction with PRORP We performed a footprinting analysis in order to map precisely contact points between a PRORP protein and its tRNA precursor substrate ( Fig. 2 ). To determine the tRNA regions that are in interaction with PRORP1, a mitochondrial tRNA Cys precursor containing a leader sequence of five nucleotides was incubated either alone or in complex with PRORP1 and subjected to digestion by nucleases. As the PRORP/tRNA complex used here was UV-crosslinked, we verified with an in vitro activity assay that substrate binding had resulted in a catalytically active complex ( Supplementary Fig. S1 ). Three different nucleases were used for this analysis, RNase V1 that only cleaves base-paired RNA regions, RNase T1 that cuts single-stranded RNA only after guanosines and RNase A that cleaves single-stranded RNA after cytidines and uridines. Positions of residues protected from RNase digestion by PRORP could be mapped down to individual nucleotides through the comparison of RNase digestion profiles with an RNase T1 ladder and the alkaline hydrolysis profile of the mitochondrial tRNA Cys precursor. We observed that discrete positions in the tRNA D-loop, namely U16, G18 and G19 were protected from nuclease digestion by PRORP. Similarly, C56 in the TψC loop was protected from nuclease digestion by PRORP. No other position, in particular close to the actual cleavage site of the tRNA precursor could be reproducibly identified as a site of nuclease protection by PRORP. Altogether, this indicates that individual residues that are in close spatial vicinity in loops D and TψC of tRNA are binding sites for protein-only RNase P enzymes ( Fig. 2 ). 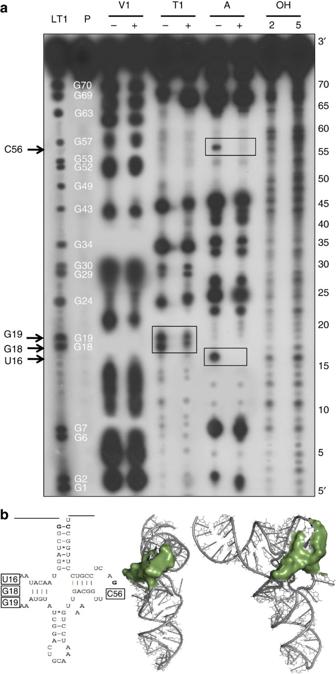Figure 2: Footprinting analysis of mitochondrial tRNACysprecursor in complex with PRORP1. (a) Samples were subjected to partial RNase V1, RNase T1 and RNase A digestions. + and − mean that PRORP proteins were present or absent in the reactions. P represents the tRNA precursor probe. LT1 shows an RNase T1 ladder with the corresponding positions of Gs in the tRNA sequence indicated in white. OH show alkaline hydrolysis of the tRNA probe performed for 2 and 5 min to generate an RNA ladder with single-nucleotide increments. RNA samples were separated by high resolution denaturing PAGE. tRNA positions were precisely mapped with the T1 and alkaline ladders. Boxed positions, also indicated on the left by arrows, correspond to tRNA positions reproducibly found protected from nuclease treatment by PRORP interaction in three replicate experiments. (b) Secondary and tertiary structural model of mitochondrial tRNACyswith boxes and green surfaces indicating residues protected by PRORP in footprinting experiments. Figure 2: Footprinting analysis of mitochondrial tRNA Cys precursor in complex with PRORP1. ( a ) Samples were subjected to partial RNase V1, RNase T1 and RNase A digestions. + and − mean that PRORP proteins were present or absent in the reactions. P represents the tRNA precursor probe. LT1 shows an RNase T1 ladder with the corresponding positions of Gs in the tRNA sequence indicated in white. OH show alkaline hydrolysis of the tRNA probe performed for 2 and 5 min to generate an RNA ladder with single-nucleotide increments. RNA samples were separated by high resolution denaturing PAGE. tRNA positions were precisely mapped with the T1 and alkaline ladders. Boxed positions, also indicated on the left by arrows, correspond to tRNA positions reproducibly found protected from nuclease treatment by PRORP interaction in three replicate experiments. ( b ) Secondary and tertiary structural model of mitochondrial tRNA Cys with boxes and green surfaces indicating residues protected by PRORP in footprinting experiments. Full size image Structural properties of PRORP 1 and 2 in solution We characterized in parallel both organellar and nuclear enzymes and focussed our study on PRORP1 and PRORP2 (which displays 80% sequence identity with PRORP3). Arabidopsis PRORP proteins are active as single-protein enzymes [9] . Their hydrodynamic properties in size exclusion chromatography and in dynamic light scattering confirmed that they are monomers in solution ( Fig. 3 ). The molecular mass determined for PRORP2 in multi-angle light scattering is 62 kDa in good agreement with that calculated from the sequence (60 kDa). 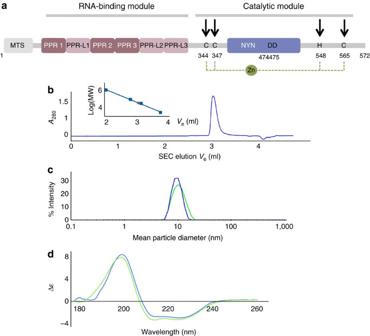Figure 3: Characterization of PRORP proteins in solution (a) Organization along the sequence of PRORP proteins. In the RNA-binding domain PPR and PPR-L show canonical PPR repeats and putative PPR-like motifs, respectively. For PRORP1, aspartates at positions 474 and 475 are in the catalytic pocket of the enzyme9, whereas cysteines and a histidine at positions 344, 347, 548 and 565 (indicated by black arrows) are proposed to form a zinc-binding pocket (dashed line) that could stabilize the catalytic domain of PRORP. (b) Analysis of PRORP2 oligomeric state in solution by analytical gel-filtration (BioSEC3 column) leading to a MW estimation of 72 kDa (red diamond: Log(MW)=4,85) by comparison with the elution of model proteins (thyroglobulin: 660 kDa; BSA monomer and dimer: 66, 132 kDa; ribonuclease A: 14 kDa; see inset). (c) Hydrodynamic radius distribution for PRORP1 (green) and PRORP2 (blue) in dynamic light scattering, confirming the monodispersity of PRORP samples. (d) SRCD analysis of PRORP1 (green) and PRORP2 (blue). SRCD spectra show a dominant peak at 190–200 nm characteristic of α-helices. The evaluation of two-dimentional structure content indicates 36/39% of α-helices, 15/16% of β-strands in PRORP1/PRORP2, respectively. Figure 3: Characterization of PRORP proteins in solution ( a ) Organization along the sequence of PRORP proteins. In the RNA-binding domain PPR and PPR-L show canonical PPR repeats and putative PPR-like motifs, respectively. For PRORP1, aspartates at positions 474 and 475 are in the catalytic pocket of the enzyme [9] , whereas cysteines and a histidine at positions 344, 347, 548 and 565 (indicated by black arrows) are proposed to form a zinc-binding pocket (dashed line) that could stabilize the catalytic domain of PRORP. ( b ) Analysis of PRORP2 oligomeric state in solution by analytical gel-filtration (BioSEC3 column) leading to a MW estimation of 72 kDa (red diamond: Log(MW)=4,85) by comparison with the elution of model proteins (thyroglobulin: 660 kDa; BSA monomer and dimer: 66, 132 kDa; ribonuclease A: 14 kDa; see inset). ( c ) Hydrodynamic radius distribution for PRORP1 (green) and PRORP2 (blue) in dynamic light scattering, confirming the monodispersity of PRORP samples. ( d ) SRCD analysis of PRORP1 (green) and PRORP2 (blue). SRCD spectra show a dominant peak at 190–200 nm characteristic of α-helices. The evaluation of two-dimentional structure content indicates 36/39% of α-helices, 15/16% of β-strands in PRORP1/PRORP2, respectively. Full size image These monodisperse PRORP samples led to sharp synchrotron radiation circular dichroism (SRCD) spectra ( Fig. 3d ) indicating that both PRORP1 and PRORP2 have a high content in α-helices. The evaluation of PRORP secondary structure content indicates 36/39% of α-helices, 15/16% of β-strands in PRORP1 / PRORP2, respectively. This observation is consistent with structure predictions based on sequence analysis [9] ( Supplementary Fig. S2 ). PRORP samples were further studied by small-angle X-ray scattering (SAXS), a method of structural characterization providing information on the size and shape of biological macromolecules in solution [19] , [20] , [21] . In these experiments, the two enzymes produced very similar scattering curves at small angles, and their estimated gyration radius is R g =33 Å corresponding to a monomer in solution ( Fig. 4 ). An experimental setup that allows the SAXS analysis downstream of a gel-filtration separation enabled the acquisition of scattering data for PRORP2 with lower noise at higher angles ( Fig. 4 , blue plot). The derived P(R) function that evaluates the distribution of distances inside the molecular object, confirms the value of R g and is compatible with an object made of two structured domains. The tail of the distribution (80< r <110 Å) suggests the presence of extension(s), which may correspond to either N-terminal or C-terminal regions. PRORP proteins are slightly more compact in solution than archaeal and bacterial RNase P RNAs, which display R g and d max of 38–48 Å and 120–190 Å in SAXS, respectively [22] , [23] . Overall, they appear as monomeric enzymes with two-domains essentially made of α-helices. 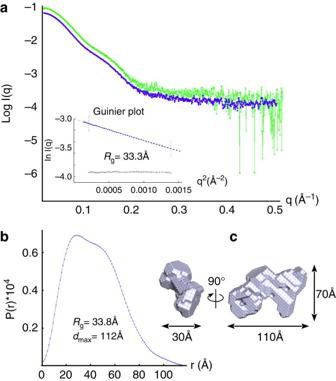Figure 4: SAXS analysis (a) PRORP1 and PRORP2 produce very similar intensity curves shown in green and blue, respectively. The inset Guinier plot indicates a gyration radius of 33.3±0.1 Å. (b) This value is confirmed by the distance distribution function P(r), which also suggests that PRORP proteins are composed of two distinct domains and an extended tail (dmax>100). (c) Molecular envelope of PRORP2 derived from SAXS data analysis. Figure 4: SAXS analysis ( a ) PRORP1 and PRORP2 produce very similar intensity curves shown in green and blue, respectively. The inset Guinier plot indicates a gyration radius of 33.3±0.1 Å. ( b ) This value is confirmed by the distance distribution function P(r), which also suggests that PRORP proteins are composed of two distinct domains and an extended tail ( d max >100). ( c ) Molecular envelope of PRORP2 derived from SAXS data analysis. Full size image PRORP proteins are zinc-binding enzymes The analysis of PRORP sequence conservation across eukaryotes revealed that a certain number of residues are highly conserved throughout evolution and might thus be of functional importance [9] . Among them, a putative zinc-finger-like structure is split in two separate motifs. The first motif (CxxC) contains two conserved cysteines upstream of the NYN domain at positions 344 and 347 for PRORP1 (281 and 284 for PRORP2), whereas the second motif involves a conserved histidine and a cysteine, downstream of the NYN domain, at positions 548 and 565, respectively, ( Fig. 3a ) (494 and 511 for PRORP2). These four particular residues were chosen as best candidates to form a zinc-binding pocket as no other cysteine or histidine outside the catalytic NYN domain is highly conserved among PRORP sequences. We used inductively coupled plasma mass spectrometry to investigate the association of metal cofactors to PRORP proteins. Zinc ( 66 Zn) was present at 29.49 +/− 1.53 p.p.b. in a 30-μg ml −1 PRORP1 solution. This corresponds to the occurrence of one zinc atom per PRORP molecule. Other metals were only found as traces. To investigate the importance of the conserved residues for zinc binding, we mutated the four residues to alanines, expressed and purified to homogeneity the respective PRORP1 mutants. The analysis of zinc content in the mutants revealed that in the C344 and C347 mutants zinc levels were reduced by 19% and 29%, respectively, whereas the H548 and the C565 mutants zinc levels decreased by 60% and 75%, respectively ( Table 1 ). As a control we analysed zinc content in the DD474-475 catalytic mutant [9] and found that it was similar to that of wild-type PRORP. The increased lability of zinc in the cysteine and histidine PRORP mutants suggests that the four residues are involved in the stable binding of zinc and that the downstream conserved motif has a stronger affinity for the metal than the upstream CxxC coordination element. We also analysed the capacity of the mutant proteins to perform RNase P activity. The single C565 mutant protein had impaired RNase P activity ( Supplementary Fig. S3 ). The highest lability of zinc in this mutant might have resulted in an unstable protein fold, thus affecting its activity. Table 1 Inductively coupled plasma mass spectrometry identifies zinc in association with PRORP. Full size table Model of the PRORP/tRNA complex Structural models of PRORP were generated by homology modelling as implemented on the Phyre server [24] . The structure prediction was limited to the two main domains (PPR and NYN) for which templates were identified with Phyre2. Best hits for the three PRORP sequences were a TPR domain (PDBid: 2ooe) and the catalytic domain of an RNase (PDB id: 3v32), respectively (see Supplementary Fig. S2 ). We also established the structure model of the Arabidopsis tRNA Cys used to illustrate footprinting experiments and activity assays. The latter data were combined with the SAXS envelope in order to position domains of PRORP2 (for which we had best SAXS data) with respect to the tRNA substrate. In the docking process, the N-terminal RNA recognition module of PRORP2 containing PPR repeats [9] was placed next to loops D and TψC of the folded tRNA, in particular in contact with positions U16, G18, G19 and C56. For the C-terminal part of the protein, the two conserved aspartates at positions 474 and 475 ( Fig. 3a ) that were shown to be part of the catalytic active site of PRORP [9] were placed in close vicinity of the tRNA +1 position, where RNase P cleavage takes place ( Fig. 5 ). Our model highlights notable similarities in tRNA-binding mode with the complex of bacterial RNP RNase P where the specificity domain of RNase P RNA interacts with the residues G19 and C56 of the tRNA ( Fig. 5 ). 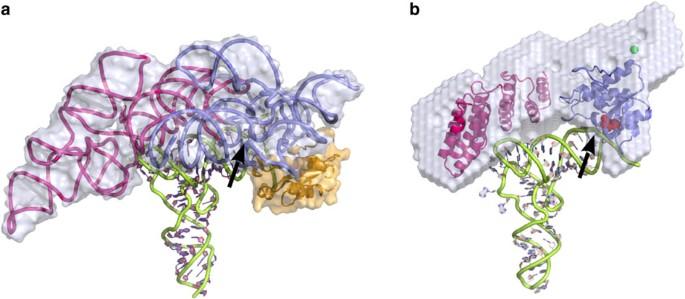Figure 5: A common mode of RNA binding in RNP and PRORP RNase P. (a) Structure ofThermotoga maritimaribozyme (PDBid 3Q1R13) with the catalytic domain in blue, the specificity domain in violet, the RNase P protein subunit in orange, the tRNA product in green and the molecular surface of the RNP in grey. (b) Model ofA. thalianaPRORP2 protein shown in the same orientation and same colour code: the catalytic domain (NYN domain) in blue, with conserved Asp residues shown as red spheres adjacent to the 5′-cleavage site (indicated by an arrow), and the RNA-binding domain (PPR domain) in violet, interacting with the region of the D-TψC loops, were positioned in the SAXS envelope. The proposed zinc site is indicated by a green sphere in the central region, which connects the two main PRORP domains. This two-domains architecture offers a concave surface, which can be docked on the tRNA acceptor arm. Our data indicate that PRORP proteins have evolved an RNA recognition process very similar to that of RNP RNase P. Figure 5: A common mode of RNA binding in RNP and PRORP RNase P. ( a ) Structure of Thermotoga maritima ribozyme (PDBid 3Q1R [13] ) with the catalytic domain in blue, the specificity domain in violet, the RNase P protein subunit in orange, the tRNA product in green and the molecular surface of the RNP in grey. ( b ) Model of A. thaliana PRORP2 protein shown in the same orientation and same colour code: the catalytic domain (NYN domain) in blue, with conserved Asp residues shown as red spheres adjacent to the 5′-cleavage site (indicated by an arrow), and the RNA-binding domain (PPR domain) in violet, interacting with the region of the D-TψC loops, were positioned in the SAXS envelope. The proposed zinc site is indicated by a green sphere in the central region, which connects the two main PRORP domains. This two-domains architecture offers a concave surface, which can be docked on the tRNA acceptor arm. Our data indicate that PRORP proteins have evolved an RNA recognition process very similar to that of RNP RNase P. Full size image PRORP enzymes were identified as members of the PPR family, a huge class of RNA-binding proteins ubiquitous in eukaryotes [25] . These proteins can be divided into two main super-groups (P and PLS) according to the occurrence of specific classes of PPR domains and of additional C-terminal domains. Several lines of evidence suggest that both types of P and PLS proteins recognize primary sequences of RNA [14] . Interestingly PRORP enzymes do not belong to the two established super-groups. With only very few canonical PPR domains, and the presence of non-canonical putative PPR repeats, they rather define a new subfamily of PPR proteins. As PRORP enzymes bind any tRNA of canonical structure, it is possible that PRORP proteins recognize structured elements of RNA and thus have a mode of RNA recognition distinct from other PPR proteins. Alternatively, our favoured hypothesis is that PPR repeats in PRORP might specifically recognize individual nucleotides in tRNA loops, in particular unstacked bases or residues not involved in Watson–Crick interactions, which are highly conserved among tRNA sequences. The biophysical characterization of PRORP enzymes has validated bioinformatic predictions and enabled to build a model of the active enzymatic complex. The predominance of SRCD signal for α-helices ( Fig. 3d ) is in agreement with fold recognition predictions, PPR repeats and NYN domains being mostly composed of α-helices [15] , [26] . Although the N-terminal region of PRORP does not contain >2–3 canonical PPR motifs, the presence of non-canonical putative PPR domains suggests that this region is arranged in a super-helix as described in structurally related TPR proteins [27] , which give the highest score in structure prediction with Phyre2. The C-terminal NYN domain could be modelled based on the structure of the MCPIP1 RNase that adopts an α–β PIN-like/NYN architecture. The Asp residues that are conserved in PRORP sequences are essential to the activity of MCPIP1 (see Supplementary Fig. S2 ) and their mutation abolished PRORP activity [9] , [28] . This observation validates the proposed fold. The region that connects the N- and C-terminal domains was identified as a potential zinc-binding motif. Our mutational analysis confirmed that the two conserved Cys residues are involved in metal binding, together with another Cys and a His residue at the C-terminal end of PRORP. Overall, this results in a compact two-domain enzyme, as confirmed by the SAXS analysis in solution, with a zinc ion bridging the central and the C-terminal region ( Fig. 5 ). Very recently, Howard and colleagues published a crystal structure of PRORP1 from A. thaliana [29] . It confirms our structural predictions, in particular the superhelical fold of the PPR domain made of 5–6 PPR and PPR-like elements. SAXS data collected in solution on PRORP1 and PRORP2 show a good agreement (experimental and theoretical curves fit with Chi of 4.9 and 2.8, respectively, for data in the range 0.02<q<0.2 Å −1 ) with the atomic model (PDB id: 4g26). This validates the overall PRORP architecture with two functional domains: a N-terminal RNA-binding PPR domain and a C-terminal PIN-like catalytic domain, bridged together by a bipartite zinc-binding module. The four residues identified by mutagenesis and inductively coupled plasma mass spectrometry as zinc binders are also confirmed by the crystal structure. Both footprint data and activity assays indicated that the tRNA precursor is essentially recognized by its acceptor arm, whereas the anticodon domain is dispensable. Results suggest that PRORP substrate recognition might be mediated by a limited number of determinants. As PRORP is able to recognize any tRNA of canonical structure, these determinants should be found among highly conserved residues such as G18 in loop D, C56 and R57 in loop TψC [30] , which is corroborated by our results. Considering the length of the acceptor arm (45 Å) and the estimation of PRORP dimensions in SAXS (30 Å × 70 Å × 110 Å), the PPR domain is very likely to interact specifically with the D-TψC region at the corner of the tRNA, while the NYN catalytic domain must be located in the vicinity of the 5′-cleavage point. Thus, the proposed model ( Fig. 5 ) shows the two-domains of PRORP2 that sandwich the substrate, their respective position acting as a ruler to determine the correct position of maturation, independently from the internal sequence of the acceptor arm. Our data suggests an intriguing similarity in the mode of binding of the tRNA with the RNP RNase P. Indeed, earlier work has shown that bacterial RNase P interaction with the D-TψC region influences substrate binding and cleavage [31] . In the same line and similar to PRORP, bacterial and human RNP RNase P did not require the anticodon domain of tRNA for substrate recognition [32] . However, E. coli RNase P, contrary to PRORP, still allowed RNase P activity on a tRNA lacking its D domain [32] . The mechanistic model of the novel protein-only RNase P represents a good basis for further investigations of PRORP mode of action by complementary approaches, the ultimate step being the determination of a crystal structure of an active complex of PRORP and tRNA at atomic resolution. The concept of structural mimicry of nucleic acids by proteins is well established, it has already been observed over 15 years ago [33] , [34] , [35] . The specific case of PRORP is particularly interesting because both a single eukaryotic protein and a considerably more ancient bacterial ribozyme share the same catalytic function and appear to share similar RNA recognition processes. This implies that PRORP could represent an example of convergent evolution, with proteins that have evolved a mechanism of RNA recognition similar to that of catalytic RNA. This opens appealing perspectives for our understanding of the transition between the envisaged pre-biotic RNA world and the modern world dominated by proteins. PRORP purification and characterization Arabidopsis recombinant PRORP1 and PRORP2 proteins were expressed in E. coli and purified to homogeneity using affinity chromatography as described previously [9] . Before biophysical analyses (see below), a second step of size exclusion chromatography using a Superdex 200 10/300 GL column (GE Healthcare) was introduced to improve the quality of PRORP enzymes and to elute them in appropriate buffers. Proteins were concentrated by ultrafiltration to about 10 mg ml −1 , ultracentrifuged and stored at 4 °C until use in 50 mM HEPES-Na pH 7.5, 250 mM NaCl, 15% glycerol (w/v), 1 mM tris (2-carboxyethyl)phosphin. Sample homogeneity and particle size were systematically verified using dynamic light scattering (Malvern Zetasizer) at 20 °C. Mass determination was performed by multi-angle light scattering using a SEC Superdex 200 column coupled to a Treos instrument (Wyatt technologies) in the storage buffer with 2% glycerol (w/v) only. RNase P activity assays cDNAs representing variants of Arabidopsis mitochondrial tRNA Cys precursors were designed with leader and trailer sequences of 50 and 30 nucleotides, respectively, cloned in pUC19, transcribed in vitro by T7 RNA polymerase. tRNA Cys precursor mutants included tRNAs with the anticodon domain removed (ΔAC), without both anticodon and D domain (ΔDAC), with point mutations at position 1, 18, 19, 56, 57 and 72. Sequences of oligonucleotide used to generate these mutants are available in Supplementary Table . For RNase P cleavage assays, reactions were always performed with three replicates using 0.5 μM transcript and 0.15 μM protein for 15 min at 25 °C as previously described [9] . RNA fragments were separated by denaturing PAGE and visualized by ethidium bromide staining. Quantifications were performed as described [10] . Footprinting analyses Recombinant PRORP1 was put in presence of equimolar amounts of 5′- 32 P-γATP radiolabeled mitochondrial tRNA Cys precursors to form a PRORP/tRNA complex. As PRORP and tRNA only interact in a transient manner, the complex obtained was UV-crosslinked for 15 min at 260 nm. Samples were submitted to partial RNase V1 (0.1 U μl −1 ), RNase T1 (1 U μl −1 ) and RNase A (1 μg μl −1 ) digestions in the presence of competitor yeast RNA according to the manufacturer’s instructions (Ambion, USA). The radiolabeled tRNA probe was also subjected to partial RNase T1 digestion in denaturing condition and to partial alkaline hydrolysis to generate RNA ladders. RNA samples were recovered by phenol/chloroform extractions, separated by high resolution 8% denaturing polyacrylamide gel electrophoresis and signal was acquired with a FLA-7000 phosphorimager (Fujifilm). SRCD analysis SRCD experiments were performed on the DISCO beamline at synchrotron SOLEIL (Saint-Aubin, France). The instrument was calibrated for magnitude and polarization with a 6.1-mg ml −1 D-10-camphorsulfonic acid solution. PRORP proteins (10 mg ml −1 ) in 100 mM potassium phosphate, 50 mM KCl, 10% (v/v) glycerol and 1 mM tris (2-carboxyethyl)phosphine were placed in a SRCD CaF 2 cuvette of 8 μm pathlength. Three spectra between 170 and 280 nm were measured at 10, 20, 30, 40, 50, 60 and 70 °C to assess the thermal stability of PRORP1 and PRORP2. Data were processed (spectrum averaging, solvent base line subtraction) using CDtools [36] . The secondary structure content of PRORPs was evaluated using the VARSLC method in DICHROWEB [37] . Small-angle X-ray scattering analysis Small-angle X-ray scattering (SAXS) experiments were conducted on the SWING beamline at Synchrotron SOLEIL, Saint-Aubin, France. The beam wavelength was set to λ =1.033 Å. The 17 × 17 cm 2 low-noise Aviex CCD detector was positioned at a distance of 2107, mm from the sample, with the direct beam off-centred. The resulting exploitable q -range was 0.005–0.5 Å −1 , where q =4 π sin θ / λ , and 2 θ is the scattering angle. PRORP samples at 10 mg ml −1 in 100 mM Hepes-Na (pH 7.5), 250 mM NaCl, 5% glycerol and 1 mM tris (2-carboxyethyl)phosphine were analysed by direct injection or high-performance liquid chromatography mode. In the first case, they were transferred into the SAXS flow-through capillary cell and a series of 50 frames was recorded. In the second case, they were loaded into a size exclusion column (Agilent Bio SEC-3, 300 Å, 4.6 × 300 mm, 3 μm) using an Agilent high-performance liquid chromatography system and eluted into the SAXS flow-through capillary cell at a flow rate of 0.2 ml min −1 . SAXS measurements were collected throughout the whole protein elution time, with a frame duration of 1000, ms and a dead time between frames of 500 ms. Data processing, analysis and modelling steps were carried out with PRIMUS [38] , and other programs of the ATSAS suite [39] . The radius of gyration R g was derived from Guinier approximation [40] and calculated from entire scattering pattern using the indirect transform package GNOM [41] , which provides the distance distribution function P(r) of the particle. Based on this distribution, ab initio modelling was carried out with DAMMIF [39] . A series of 11 dummy atom models was generated that were compared using the DAMAVER suite [42] to determine the most typical/probable one (that is, showing the lowest averaged normalized spatial discrepancy). The molecular envelope corresponding to this model was used to spatially restrain the positions of PRORP domains and of the tRNA substrate in the model. Inductively coupled plasma mass spectrometry For the (w/v) analysis of metal cofactors, PRORP solutions resuspended in 0.5 N nitric acid were analysed with a ThermoElectron X Series II inductively coupled plasma mass spectrometry mass spectrometer operated at 1450 W, with argon carrier gas flow rate of 0.85 l min −1 , argon auxiliary gas flow rate of 0.40 l min −1 , using a Meinarht quarz nebulizer, a quarz spray chamber with impact bead chilled to 3 °C and sample flow rate set to 0.1 l min −1 . Four replicate measurements were performed and values were corrected by an internal 115 In standard. Structure modelling The overall architecture of PRORP domains was predicted by homology modelling based on the alignment of 181 PRORP ortholog sequences [9] and fold recognition to find remotely related candidates with known structure as implemented on the Phyre2 server [24] . PRORP RNA partner (pre-tRNA Cys from A. thaliana ) was modelled using S2S [43] based on a sequence alignment with the tRNA Cys from E. coli (PDB-id 1B23 [44] ). PRORP domain models were fit in the SAXS envelope and the tRNA substrate was docked on its concave surface in a way bringing the PPR and catalytic domains in close vicinity of the D-TψC corner and of the cleavage point, respectively. Molecular docking and related figures were performed with PyMOL (The PyMOL Molecular Graphics System, Version 1.5.0, Schrödinger, LLC). How to cite this article: Gobert, A. et al. Structural insights into protein-only RNase P complexed with tRNA. Nat. Commun. 4:1353 doi: 10.1038/ncomms2358 (2013).